Nucleoporin 107, 62 and 153 mediateKcnq1ot1imprinted domain regulation in extraembryonic endoderm stem cells Genomic imprinting is a phenomenon that restricts transcription to predominantly one parental allele. How this transcriptional duality is regulated is poorly understood. Here we perform an RNA interference screen for epigenetic factors involved in paternal allelic silencing at the Kcnq1ot1 imprinted domain in mouse extraembryonic endoderm stem cells. Multiple factors are identified, including nucleoporin 107 (NUP107). To determine NUP107’s role and specificity in Kcnq1ot1 imprinted domain regulation, we deplete Nup107 , as well as Nup62, Nup98/96 and Nup153 . Nup107 , Nup62 and Nup153 , but not Nup98/96 depletion, reduce Kcnq1ot1 noncoding RNA volume, displace the Kcnq1ot1 domain from the nuclear periphery, reactivate a subset of normally silent paternal alleles in the domain, alter histone modifications with concomitant changes in KMT2A, EZH2 and EHMT2 occupancy, as well as reduce cohesin interactions at the Kcnq1ot1 imprinting control region. Our results establish an important role for specific nucleoporins in mediating Kcnq1ot1 imprinted domain regulation. Genomic imprinting is an epigenetic process that restricts expression of specific genes to predominantly the maternally- or paternally inherited allele. The biochemical mechanisms that generate this allele-specific asymmetry rely upon multiple protein families, broadly termed epigenetic factors. However, it is still not fully clear which specific epigenetic factors establish and maintain this duality. In this study, we investigated the Kcnq1ot1 domain to further understand the mechanisms involved in allele-specific asymmetry. The Kcnq1ot1 domain serves as an excellent model of imprinted domain regulation, since all known epigenetic regulatory mechanisms have some role at the Kcnq1ot1 imprinted domain, including differential DNA methylation and chromatin modifications, noncoding RNA expression, transcriptional interference, noncoding RNA-mediated silencing, CCCTC-binding factor (CTCF)/cohesin insulator activity and chromatin looping [1] , [2] , [3] , [4] , [5] , [6] , [7] , [8] , [9] . Within the Kcnq1ot1 domain resides the imprinting control region (ICR), the paternally expressed Kcnq1ot1 ( Kcnq1 opposite transcript 1) noncoding RNA (ncRNA), 9 maternally expressed protein-coding genes, and several genes that escape imprinting [1] , [4] , [8] , [10] , [11] . On the maternal allele, the Kcnq1ot1 ICR is methylated, silencing the embedded Kcnq1ot1 promoter and its transcription, thereby permitting expression of neighboring genes. On the paternal allele, the Kcnq1ot1 ICR is unmethylated, allowing Kcnq1ot1 ncRNA transcription, which results in protein-coding gene silencing. In mice, paternal inheritance of a Kcnq1ot1 ICR deletion leads to paternal reactivation of imprinted genes within the domain at midgestation [12] . Similarly, paternal transmission of Kcnq1ot1 ncRNA truncations result in paternal allelic reactivation in midgestation embryos [5] , [6] . These results indicate that the Kcnq1ot1 ICR as well as Kcnq1ot1 ncRNA/transcription are essential for paternal allelic silencing. To date, several epigenetic factors have been identified that regulate Kcnq1ot1 domain imprinting, including polycomb repressive complex (PRC) 1 and 2 proteins (E3 ubiquitin-protein ligase RING2 (RNF2), enhancer of zeste homolog 2 (EZH2), embryonic ectoderm development (EED)), histone methyltransferase 2 (EHMT2/G9a), suppressor of variegation 4-20 homolog 1 (SUV420H1) and DNA methyltransferase 1 (DNMT1) [3] , [8] , [9] , [13] , [14] , [15] , [16] . Here, we identify multiple epigenetic factors involved in Kcnq1ot1 imprinted domain regulation, including a nucleoporin-dependent mechanism. We show that NUP107, NUP62, and NUP153 are required in extraembryonic endoderm stem cells to maintain Kcnq1ot1 ncRNA expression and volume at the domain, to position the Kcnq1ot1 imprinted domain at the nuclear periphery, as well as to silence a subset of paternal alleles of the protein-coding genes in the domain. We also show that nucleoporins regulate imprinted gene expression through active and repressive histone modifications but not DNA methylation at the ICR. Lastly, we show nucleoporins direct the occupancy of cohesin complex proteins at the paternal Kcnq1ot1 ICR. Multiple epigenetic factors silence a paternal NeoR cassette To identify epigenetic factors involved in paternally inherited NeoR silencing, as a proxy for paternal allelic silencing of imprinted genes in the Kcnq1ot1 domain, a positive-selection, loss-of-function RNA interference screen was performed using a library of short hairpin RNAs (shRNAs) for 250 epigenetic factors, with ~3 hairpins per factor [17] (Supplementary Fig. 1 ). To conduct this screen, we used an existing transgenic mouse model, where exons 1 and 2 of the Cdkn1c imprinted gene were replaced with the PGK-neomycin resistance cassette ( Cdkn1c +/ΔneoR ) [18] (Supplementary Fig. 2a ). Our strategy was predicated upon silencing of the paternally inherited drug resistance marker ( Cdkn1c ΔneoR ) [19] in CAST7XB6 Cdkn1c +/ΔneoR embryonic, trophoblast and extraembryonic endoderm (XEN) stem cells. Reactivation of the silent Cdkn1c ΔneoR allele following depletion allowed for survival and selection of colonies in the presence of neomycin, and thus, identification of epigenetic factors crucial in maintaining its silent state. Albeit, only XEN cells displayed repression of the paternally inherited Cdkn1c ΔneoR allele to a level that would allow efficient screening (Supplementary Fig. 2b ). Using this strategy, 696 colonies were picked for a second round of neomycin selection, following which 297 colonies were isolated. DNA was sequenced to identify shRNA-targeted factors controlling Cdkn1c ΔneoR repression (Supplementary Fig. 1 ). 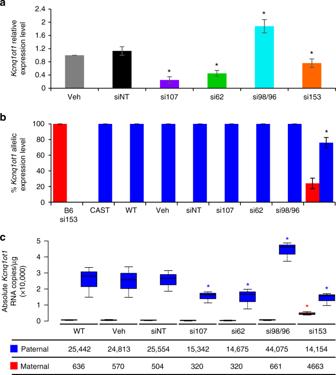Fig. 1 Nucleoporin depletion disruptedKcnq1ot1ncRNA expression.aReal-timeKcnq1ot1 ncRNA expression levels normalized toGapdh(n= 3 biological samples with four technical replicates per sample).bAllelicKcnq1ot1ncRNA expression in control andNup-depleted XEN cells (n= 3 biological samples;n= 4 technical replicates per sample).cAbsolute allelicKcnq1ot1 transcript abundance determined by droplet digital PCR in control andNup-depleted XEN cells, as measured by RNA copies µg−1(n= 3 biological samples). Center lines, medians; box limits, 25th and 75th percentiles as determined by R software; whiskers, 1.5 times the interquartile range from 25th and 75th percentiles; B6/maternal, red; CAST/paternal, blue; error bars, s.e.m.; *, significancep< 0.05 compared to siNT control (ttest); WT wild type, Veh vehicle, siNT nontargeting siRNA, si107Nup107siRNA, si62Nup62siRNA, si98/96Nup98/96siRNA, si153Nup153siRNA In total, 41 epigenetic modifiers were identified (Table 1 ), with stronger candidates having multiple independent colonies and hairpins recovered. Candidates included factors (RNF2, EZH2, EED, SUV420H1, and DNMT1) previously shown to play a role in Kcnq1ot1 imprinted domain regulation [3] , [7] , [9] , [13] , [14] , [15] , [16] , [20] , validating our screening strategy. However, they were recovered at a lower frequency than other candidates. Given the chance of off-target effects, validation of candidates will be required to delineate their role in paternal allelic silencing at the Kcnq1ot1 domain. Here, we focused on the candidate nucleoporin 107 ( Nup107 ) (Table 1 ). Nucleoporins are proteins that constitute nuclear pore complexes that stud the nuclear membrane, allowing nuclear-cytoplasmic transport [21] . A more recent role identified for nucleoporins is gene regulation, although the mechanistic underpinnings of this regulation are not fully understood [22] , [23] , [24] , [25] , [26] , [27] , [28] . Table 1 Candidate epigenetic factors of the Kcnq1ot1 imprinted domain Full size table Nucleoporins regulate Kcnq1ot1 ncRNA expression and volume To investigate the role and specificity of NUP107, we examined NUP107, as well as three additional nucleoporins with documented chromatin association [23] , [27] , [28] (NUP62, NUP98 and NUP153, not included in our original screen) for their role in regulating the Kcnq1ot1 imprinted domain. B6XCAST XEN cells were transfected with two sets of Nup107 , Nup62 , Nup98/96 and Nup153 siRNAs to produce RNA and protein depletion (Supplementary Fig. 3a–d , antibody validation; Supplementary Fig. 4a, b ). Cells were then assessed for total and allele-specific Kcnq1ot1 ncRNA expression. Compared to controls, Nup107 , Nup62 and Nup153 depletion significantly reduced Kcnq1ot1 ncRNA levels to 0.25, 0.45 and 0.76 of controls, respectively, while Nup98/96 depletion produced a 1.88 times increase in Kcnq1ot1 ncRNA levels (Fig. 1a ). For all Nup depletions, the Kcnq1ot1 ncRNA maintained paternal expression (Fig. 1b ), except for Nup153 depletion, where the normally silent maternal Kcnq1ot1 ncRNA was reactivated (24%). To determine absolute maternal and paternal expression levels instead of allelic ratios, we developed a highly sensitive, precision method for assessing absolute transcript abundance of each allele independently using droplet digital PCR with FAM and HEX strain-specific probes (Supplementary Fig. 5 ). Compared to control cells, there was a significant decrease in paternal Kcnq1ot1 transcripts by 9928-11,116 copies upon Nup107 , Nup62 , and Nup153 depletion, and a significant increase in paternal Kcnq1ot1 transcripts by 18,805 copies upon Nup98/96 depletion (Fig. 1c ). While Nup107 , Nup62 , and Nup98/96 depletion did not change the low number of maternal Kcnq1ot1 transcripts, Nup153 depletion produced a significant increase in maternal Kcnq1ot1 transcripts by 4093 copies, compared to controls. Fig. 1 Nucleoporin depletion disrupted Kcnq1ot1 ncRNA expression. a Real-time Kcnq1ot 1 ncRNA expression levels normalized to Gapdh ( n = 3 biological samples with four technical replicates per sample). b Allelic Kcnq1ot1 ncRNA expression in control and Nup -depleted XEN cells ( n = 3 biological samples; n = 4 technical replicates per sample). c Absolute allelic Kcnq1ot 1 transcript abundance determined by droplet digital PCR in control and Nup -depleted XEN cells, as measured by RNA copies µg −1 ( n = 3 biological samples). Center lines, medians; box limits, 25th and 75th percentiles as determined by R software; whiskers, 1.5 times the interquartile range from 25th and 75th percentiles; B6/maternal, red; CAST/paternal, blue; error bars, s.e.m. ; *, significance p < 0.05 compared to siNT control ( t test); WT wild type, Veh vehicle, siNT nontargeting siRNA, si107 Nup107 siRNA, si62 Nup62 siRNA, si98/96 Nup98/96 siRNA, si153 Nup153 siRNA Full size image Paternal Kcnq1ot1 ncRNA transcripts coat the paternal Kcnq1ot1 domain in what is thought to be a repressive nuclear compartment [8] , [11] , [15] , [29] . To determine whether reduced Kcnq1ot1 ncRNA abundance altered nuclear Kcnq1ot1 ncRNA volume, 3D Kcnq1ot1 RNA/DNA FISH was performed on G1-synchronized control and Nup -depleted XEN cells, and Kcnq1ot1 ncRNA volume was calculated. Kcnq1ot1 ncRNA signal was restricted to the paternal Kcnq1ot1 domain in controls, with a reduction in cells with paternal Kcnq1ot1 ncRNA signal in Nup107- , Nup62- , and Nup153- but not Nup98/96 -depleted XEN cells (Fig. 2a, b ). Nup153 -depleted XEN cells also displayed Kcnq1ot1 ncRNA signal at the maternal domain in 32% of cells. With respect to Kcnq1ot1 ncRNA volume, the majority of control cells possessed medium volumes (70–72%; low, 13–18%; high, 11–15%; very high, 0–1%) (Fig. 2d ). Consistent with altered Kcnq1ot1 ncRNA levels, Nup107 , Nup62 , and Nup153 depletion generated a significant increase in cells with low Kcnq1ot1 ncRNA volumes (83, 76, 26%, respectively), while Nup98/96 depletion significantly increased the number of cells with high (35%) or very high (15%) volumes (Fig. 2d ). In addition, upon Nup153 depletion, 76% of cells with maternal Kcnq1ot1 reactivation had low Kcnq1ot1 ncRNA volumes. Notably, changes in Kcnq1ot1 ncRNA abundance and volume were not due to altered Kcnq1ot1 transcript stability (Supplementary Fig. 6 ). Together, these results demonstrate that nucleoporins facilitate paternal Kcnq1ot1 ncRNA expression. Fig. 2 Nucleoporin depletion disrupted Kcnq1ot1 ncRNA volume and Kcnq1ot1 domain positioning at the nuclear periphery. a Representative confocal nuclear images displaying Kcnq1ot1 DNA (magenta) Kcnq1ot1 ncRNA (cyan) and DAPI staining (blue) for G1-synchronized control and Nup -depleted XEN cells ( n = 4; cell number = 109–123); upper panel, DNA FISH; middle panel, RNA FISH; lower panel, merge; M maternal domain, P paternal domain; white dashed line denotes nuclear rim. In these images, red and green fluorescence was converted to magenta and cyan. b , c Percent of cells with paternal or maternal Kcnq1ot1 ncRNA signals. d Percent of cells with Kcnq1ot1 ncRNA signal volume; low, 0–0.7 μm 3 ; medium, 0.7–1.4 μm 3 ; high, 1.4–2.1 μm 3 ; very high, >2.1 μm 3 . e Distance of the paternal and maternal Kcnq1ot1 domain from the nuclear membrane in control and Nup -depleted XEN cells. The maternal Kcnq1ot1 domain was randomly positioned within the nucleus (expected nuclear periphery (NP) 15%; subnuclear periphery (SP) 30%; nuclear interior (NI) 60%), except for Nup153 -depleted cells with a Kcnq1ot1 ncRNA signal (si153 M+). For these analyses, cells with no RNA but detectable DNA FISH signals were included, while those lacking DNA signals were excluded. NP, 0–0.5 μm; SP, 0.5–1.5 μm; NI, 1.5–4 μm; error bars, s.e.m. ; *, significance p < 0.05 compared to vehicle control ( t test); WT wild type, Veh vehicle, siNT nontargeting siRNA, si107 Nup107 siRNA, si62 Nup62 siRNA, si98/96 Nup98/96 siRNA, si153 Nup153 siRNA, si153 M- Nup153 -depleted cells without a Kcnq1ot1 ncRNA signal; scale bar, 1 μm; n = 4; cell count number = 109–123 Full size image NUPs position the Kcnq1ot1 domain to the nuclear periphery Previous studies demonstrated that the Kcnq1ot1 ncRNA-coated domain can be situated at the nuclear periphery [7] , [8] , and that the distance between distal probes within the Kcnq1ot1 domain differed for maternal and paternal alleles [11] , [15] . To examine the position of the Kcnq1ot1 domain in XEN cells, distance of the Kcnq1ot1 DNA signal centroid from the nuclear rim was calculated [30] , [31] . Here, size of the Kcnq1ot1 DNA volume identified the maternal (0.1–0.8 μm 3 ) and paternal (0.9–1.3 μm 3 ) domains (Supplementary Fig. 7 ). In control cells, the paternal Kcnq1ot1 domain was stationed at the nuclear periphery, subnuclear periphery and nuclear interior in 92, 4–6, and 3–4% of cells, respectively (Fig. 2e ). In Nup107- , Nup62- and Nup153- depleted XEN cells, nuclear periphery positioning of the paternal Kcnq1ot1 domain was significantly reduced to 54, 61, and 64% of the cells, shifting to the subnuclear periphery (26, 33, and 17%) and nuclear interior (20, 6, and 19%), respectively. Furthermore, maternal Kcnq1ot1 domain positioning was significantly increased at the nuclear periphery in Nup153- depleted XEN cells possessing a maternal Kcnq1ot1 ncRNA signal (+; 60%) compared to control cells (14–17%) and Nup153- depleted XEN cells without a maternal Kcnq1ot1 ncRNA signal (−; 9%). Nup98/96 depletion also significantly reduced paternal Kcnq1ot1 domain nuclear peripheral (84%) positioning, albeit to a lesser extent than other Nup depletions. Next, we examined the relationship between Kcnq1ot1 ncRNA volume and nuclear positioning. The majority of control cells had medium paternal Kcnq1ot1 ncRNA volume that resided at the nuclear periphery (Supplementary Fig. 8 ). By comparison, in Nup107- and Nup62 -depleted cells with low paternal Kcnq1ot1 ncRNA volume, the Kcnq1ot1 domain was displaced from the nuclear periphery. In Nup153 -depleted cells, paternal Kcnq1ot1 domains with low and medium Kcnq1ot1 ncRNA volumes shifted away from the nuclear periphery, while maternal domains with low and medium Kcnq1ot1 ncRNA volumes shifted toward the nuclear periphery. In contrast, Nup98/96 -depleted cells with increased paternal Kcnq1ot1 ncRNA volumes primarily retained nuclear peripheral positioning of the Kcnq1ot1 domain. These results indicate that NUP107, NUP62, and NUP153 target the Kcnq1ot1 ncRNA-coated domain to the nuclear periphery. NUPs bind the Kcnq1ot1 ICR and imprinted gene promoters We next investigated nucleoporin interactions with the Kcnq1ot1 imprinted domain. Quantitative chromatin immunoprecipitation (ChIP) was performed using mAb414 (primarily interacts with NUP62, NUP107, and NUP160 in XEN cells (Supplementary Fig. 3b )) and NUP153 antibodies; ChIP-grade NUP107 and NUP62 antibodies were not available. Antibodies were first validated at predictive positive and negative sites identified from mouse ES cells NUP153 DNA adenine methyltransferase identification sequencing (DamID-seq) data [27] (Supplementary Fig. 9 ). To investigate nucleoporin interactions at the Kcnq1ot1 domain, 21 sites across the Kcnq1ot1 ICR through to the reported H3K4me1-enriched enhancer element [32] , [33] , 1–2 sites at imprinted gene promoters, and two control regions were assessed for total and allele-specific binding in WT XEN cells (Supplementary Fig. 10a , Fig. 3a ). Significant mAb414 (NUP107/62) enrichment was observed at two sites within the Kcnq1ot1 ICR (IC3, 100 bp upstream; IC4, 1.7 kb downstream of the Kcnq1ot1 transcription start site), the Kcnq1ot1 enhancer element (E1 and E2) and the Osbpl5 promoter (Os1 and Os2) on the paternal allele (Supplementary Fig. 10b , Fig. 3b, d ). Significant NUP153 enrichment was observed at the Kcnq1ot1 ICR (IC3, IC4), where both parental alleles were equally enriched, and at the paternal Kcnq1 (Kc1, Kc2) and Cd81 (Cd1) promoters (Supplementary Fig. 10b , Fig. 3c, e ). By comparison, no NUP98 enrichment was observed at the Kcnq1ot1 ICR or enhancer element (Supplementary Fig. 10b ). Next, we investigated whether nucleoporin−chromatin interactions were lost upon Nup depletion. Since the mAb414 antibody recognizes NUP62 and NUP107 (Supplementary Fig. 3b ), double depletion was performed. We found a significant decrease in nucleoporin occupancy at the Kcnq1ot1 ICR and enhancer element in double-depleted cells at the paternal allele (Fig. 3d ). Upon Nup153 depletion, NUP153 binding on the paternal and maternal Kcnq1ot1 ICR, and the paternal Kcnq1 and Cd81 promoters was significantly reduced (Fig. 3e ). To determine whether there was interdependency between NUP107/62 and NUP153 binding, Nup153- depleted cells were examined for mAb414 enrichment, and Nup107- and Nup62- depleted cells were assessed for NUP153 enrichment. Nup153 depletion significantly decreased mAb414 (NUP107/62) binding at the Kcnq1ot1 ICR region but not at the Osbpl5 promoter and enhancer sites (Fig. 3f ). Conversely, Nup107 and Nup62 depletion significantly decreased NUP153 occupancy at the Kcnq1ot1 ICR and Kcnq1 promoter, while no change in enrichment was observed at the Cd81 promoter (Fig. 3g ). These results indicate that nucleoporin interactions at the paternal Kcnq1ot1 ICR are cooperatively mediated through NUP107/NUP62 and NUP153. Fig. 3 NUP107/62 and NUP153 interaction with the Kcnq1ot1 ICR, and the Osbpl5, Kcnq1, Cd81 promoters. a The Kcnq1ot1 domain with regions of analysis (arrowheads) at the Kcnq1ot1 ICR, IC3, IC4; enhancer element, E1, E2; imprinted gene promoters; Os1, Os2, Ph1, Ph2, Sl1, Sl2, Ck1, Kc1, Kc2, Ts1, Ts2, Cd1, Th1; and negative control sites, Ctrl1, Ctrl2. Quantitative ChIP analysis using b mAb414 antibodies and c NUP153 antibodies in wild-type XEN cells at regions across the domain, respectively ( n = 3 biological samples with four technical replicates per sample). Quantitative allelic analysis for d mAb414 and e NUP153 in siNT- and nucleoporin-depleted XEN cells. Allelic proportions are represented as percent of the total enrichment levels ( n = 3 biological samples with four technical replicates per sample). f Quantitative ChIP analysis using mAb414 antibodies was performed in control and Nup153 -depleted XEN cells at sites of NUP153 enrichment ( n = 3 biological samples with three technical replicates per sample). g Quantitative ChIP analysis using NUP153 antibodies was performed in control and Nup107- and Nup62- depleted cells at sites of mAb414 (NUP107/62) enrichment ( n = 3 biological samples with three technical replicates per sample). Error bars, s.e.m. ; *, significance p < 0.05 compared to the IgG or siNT control ( t test) Full size image We further investigated whether nucleoporins can interact with a Kcnq1ot1 ICR DNA fragment in nuclear lysates from control and Nup -depleted XEN cells. Electromobility shift assays were first performed using biotin-labeled Vim , Shank2 and Dchr7 promoter fragments as controls. For the Kcnq1ot1 , supershifts were observed for the biotin-labeled Kcnq1ot1 ICR fragment with mAb414 (NUP107/62), NUP107, and NUP153 antibodies but not for the biotin-labeled, 2-kb upstream control fragment (Supplementary Fig. 11a, b ), pointing to a direct interaction of these proteins with the Kcnq1ot1 ICR. No supershift was produced using the NUP98 antibody. Next, reverse ChIP was performed to isolate proteins bound to a biotin-labeled Kcnq1ot1 ICR and negative control fragments, followed by western blot analysis using NUP107, mAb414, NUP98, and NUP153 antibodies. NUP107 bound to the Kcnq1ot1 ICR fragment but not the 2-kb upstream control fragment (Supplementary Fig. 12 ). Nup107 -depleted lysates abrogated NUP107 binding, as well as NUP62 and NUP153 binding, indicating that NUP62 and NUP153 binding at the Kcnq1ot1 ICR required NUP107 binding. NUP153 also bound directly to the Kcnq1ot1 ICR fragment but not the control fragment. Upon Nup153 depletion, binding to the Kcnq1ot1 ICR fragment was lost, although NUP107 and NUP62 binding was not altered, perhaps indicating sequential binding of NUP107, NUP62, and NUP153. NUPs regulate paternal allelic silencing of imprinted genes Since NUP107, NUP62, and NUP153 were bound within the Kcnq1ot1 domain, allelic expression of imprinted genes in the Kcnq1ot1 domain was assessed by a conventional method of allelic ratio quantification [1] . Nup107 , Nup62 , and Nup153 depletion resulted in paternal reactivation of the core group of genes, Slc22a18 , Cdkn1c , and Kcnq1 (Supplementary Fig. 13 ), as well as gene-specific reactivation (paternal Osbpl5 and Phlda2 alleles upon Nup107 depletion, the paternal Osbpl5 allele upon Nup62 depletion, and the paternal Cd81 allele upon Nup62 depletion). By comparison, Nup98/96 depletion had no effect on paternal allelic expression. To determine the absolute transcript abundance of maternal and paternal RNA copies, we developed allelic droplet digital PCR assays using FAM and HEX strain-specific probes for imprinted genes in the domains (Fig. 4 , Supplementary Fig. 14 ). Compared to controls, we observed that Nup107 and Nup62 depletion increased paternal Osbpl5 transcripts by 13,472–13,662 copies, Nup107 depletion increased Phlda2 transcripts by 430 copies, Nup107, Nup62 , and Nup153 depletion increased paternal transcripts of Slc22a18 by 29,547–32,214, Cdkn1c by 10,882–13,153, and Kcnq1 by 728–805 copies, and Nup153 depletion increased Cd81 transcripts by 13,033 copies (Fig. 4 , Supplementary Fig. 15 ). Notably, even though the normally silent maternal Kcnq1ot1 allele was reactivated in a proportion of Nup153 -depleted XEN cells, no change was observed in maternal transcript copies of imprinted genes upon Nup153 depletion. Overall, our data indicate that paternal allelic reactivation was not domain-wide. Instead, NUP107, NUP62, and NUP153 regulate paternal allelic silencing of a core group of genes, Slc22a18 , Cdkn1c , and Kcnq1 , while paternal allele silencing of genes more distal to the Kcnq1ot1 ICR, Phlda2 , Osbpl5, and Cd81 , was nucleoporin-specific. Fig. 4 Nup107, Nup62 , and Nup153 depletion reactivate a subset of paternal alleles at the Kcnq1ot1 domain. Absolute allelic transcript abundance of imprinted genes determined by droplet digital PCR in control and Nup -depleted XEN cells, as a measure of RNA copies µg −1 ( n = 3 biological samples). Center lines, medians; box limits, 25th and 75th percentiles as determined by R software; whiskers, 1.5 times the interquartile range from 25th and 75th percentiles; Mat, maternal; Pat, paternal; Pat R, reactivated paternally silent allele; *, significance p < 0.05 compared to the siNT control ( t test). Error bars, s.e.m. Full size image Nuclear-cytoplasmic transport not impaired by Nup depletion An alternate explanation for altered regulation of the Kcnq1ot1 domain upon nucleoporin depletion is impaired nuclear-cytoplasmic transport. The nuclear pore complex is composed of multiple copies of ~30 nucleoporins (~500 proteins in total) [34] . Impaired function may result from incorrect assembly of the nuclear pore complex when one component is depleted. Examining the levels of various nucleoporins within different structural components of the nuclear pore (Supplementary Fig. 16a ), we found no change in nucleoporin levels in Nup -depleted XEN cells compared to controls (Supplementary Fig. 16b ), suggesting that nuclear pore complex assembly was not affected upon Nup depletion. Previous studies have shown that import of cargo containing a classical bipartite nuclear localization signal (NLS) was impaired in NUP153 -depleted HeLa cells [35] . We found no change in protein import in control and Nup -depleted XEN cells as measured by levels of the transcription factor 3 (E47)-red fluorescence protein (RFP)-NLS construct [36] compared to ivermectin-treated cells, where RFP import was inhibited (Supplementary Fig. 17a ), or between endogenous inner centromeric protein (INCENP) levels (Supplementary Fig. 17b ) or LAMINB1 protein localization (Supplementary Fig. 17c ). With respect to export, previous studies found aberrant nuclear mRNA export in NUP107 -depleted HeLa cells, with abnormal accumulation of polyA-mRNA in depleted nuclei [37] . Here, no significant difference in nuclear polyA-mRNA retention levels was observed between control and Nup -depleted XEN cells (Supplementary Fig. 17d ). With regard to passive bidirectional diffusion, we found that Nup -depleted cells exhibited comparable levels of nuclear and cytoplasmic GFP mRNA as well as nuclear GFP protein from a Luciferase gene tagged with a GFP reporter protein (shLucGFP) [17] , [38] , [39] (Supplementary Fig. 17e ). Since aberrant nuclear transport may be expected to compromise cellular function [37] , a final test was conducted to measure XEN cell growth rate. No significant change in XEN cell growth rate or doubling time was observed in control and Nup -depleted XEN cells in a direct cell counting assay (Supplementary Fig. 18a, b ), which was similar to NUP107 -depleted HeLa cells [37] . Overall, these results indicate that nuclear-cytoplasmic transport in XEN cells was not affected by nucleoporin depletion. DNA methylation not altered by Nup depletion Another explanation for a reduction in paternal Kcnq1ot1 ncRNA levels and subsequent paternal allelic reactivation upon Nup107, Nup62 , and Nup153 depletion could be a gain of DNA methylation at the normal unmethylated paternal ICR. In addition, reactivation of maternal Kcnq1ot1 in Nup153 -depleted XEN cells could be explained by a loss of DNA methylation at the methylated maternal ICR. Analysis of parental-specific methylation demonstrated that the maternal Kcnq1ot1 ICR was hypermethylated while the paternal ICR was hypomethylated in control and Nup -depleted XEN cells (Supplementary Fig. 19 ). Thus, changes in NUP107, NUP62, and NUP153 regulation at the Kcnq1ot1 imprinted domain were not through alterations in Kcnq1ot1 ICR methylation. NUPs maintain chromatin at Kcnq1ot1 ICR and gene promoters We next investigated whether altered Kcnq1ot1 ncRNA expression and paternal allelic silencing at the Kcnq1ot1 imprinted domain is due to alterations in chromatin state [4] , [9] , [15] , [40] . ChIP assays were performed on control and depleted XEN cells using antibodies directed against RNAPII and histone 3 lysine 4 trimethylation (H3K4me3) as marks for active chromatin, and H3K9me2 and H3K27me3 for repressed chromatin. H3K4me3 and H3K27me3 peaks in XEN cells were used for primer placement [41] . Antibodies were first validated at the XEN cell expressed FoxA2 gene and XEN cell repressed MyoD gene [17] , [42] , where active and repressive modifications were observed, respectively (Supplementary Fig. 20 ). At the Kcnq1ot1 domain, we first verified equal allelic detection in input chromatin (Supplementary Fig. 21 ) as well as equivalent enrichment for histone 3 (H3), a protein expected on both parental alleles (Supplementary Fig. 22 ). For the Kcnq1ot1 ICR, there was a significant decrease in RNAPII and H3K4me3 enrichment and a significant increase in H3K9me2 and/or H3K27me3 enrichment on the paternal Kcnq1ot1 ICR in Nup107- , Nup62 -, and Nup153 -depleted cells compared to control cells (Fig. 5a, b ), which would account for reduced paternal Kcnq1ot1 ncRNA levels. In addition, on the maternal Kcnq1ot1 ICR, we observed a significant increase in H3K4me3 and RNAPII enrichment along with decreased repressive histone modifications upon Nup153 depletion, which could account for reactivation of the maternal transcript. At the promoters of imprinted genes in the domain, there was significantly increased enrichment of RNAPII and/or H3K4me3 at the paternal Slc22a18 , Cdkn1c, and Kcnq1 alleles upon Nup107 , Nup62 , and Nup153 depletion, at the paternal Osbpl5 and Phlda2 promoters upon Nup107 and Nup62 depletion, and at the paternal Cd81 promoter upon Nup153 depletion compared to control cells (Fig. 5a, b ). This corresponded with significantly reduced levels of H3K9me2 and/or H3K27me3, thereby accounting for their paternal reactivation. No significant changes in histone modifications were observed upon Nup98/96 depletion (Fig. 5a, b ). These results demonstrate that NUP107, NUP62, and NUP153 act to regulate histone modifications at the Kcnq1ot1 ICR and at specific imprinted gene promoters. Fig. 5 Nup107, Nup62 , and Nup153 depletion disrupts RNAPII enrichment and histone modifications at the Kcnq1ot1 ICR and imprinted gene promoters. a RNAPII and H3K4me3 ChIP at the maternal and paternal Kcnq1ot1 ICR and imprinted gene promoters in control and Nup -depleted XEN cells ( n = 3; n = 3 technical replicates). b H3K9me2 and H3K27me3 ChIP at the maternal and paternal Kcnq1ot1 ICR and imprinted gene promoters in control and Nup -depleted XEN cells ( n = 3 biological samples with three technical replicates per sample). The y -axis indicates total and allelic ChIP enrichment levels represented as percent of input. Allelic proportions are represented as a percent of the total ChIP enrichment level. Error bars, s.e.m. ; *, significance p < 0.05 of paternal/maternal levels compared to the siNT paternal/maternal control ( t test) Full size image Changes in histone modifications could be a consequence of altered histone methyltransferases or RNAPII binding at the Kcnq1ot1 ICR and imprinted gene promoters upon nucleoporin depletion. First, we ruled out that nucleoporin depletion per se did not alter histone 3 lysine 4 methyltransferase 2a (KMT2A), EHMT2, EZH2, and RNAPII protein levels in control and Nup -depleted XEN cells (Supplementary Fig. 23a, b ). We found decreased KMT2A, and increased EHMT2 and EZH2 enrichment levels upon Nup107/62 and Nup153 depletion compared to control and Nup98/96 -depleted cells (Fig. 6a–c ). At imprinted gene promoters with altered histone modifications, KMT2a enrichment was increased on the paternal Osbpl5 , Phlda2 , Slc22a18 , Cdkn1c , and Kcnq1 alleles upon Nup107/62 depletion, and on the paternal Slc22a18 , Cdkn1c , Kcnq1 , and Cd81 alleles upon Nup153 depletion, while a corresponding decrease in EHMT2 and EZH2 recruitment was found on the paternal Osbpl5 , Cdkn1c , Kcnq1 , and Cd81 alleles upon Nup107/62 and/or Nup153 depletion. Surprisingly, no change in EHMT2 and EZH2 levels were observed at the Slc22a18 promoter. Overall, these results suggest that changes in H3K4me3, H3K9me2, and H3K27me3 levels were conferred by alteration in KMT2A, EHMT2, and EZH2 binding, respectively, at the Kcnq1ot1 ICR and imprinted gene promoters upon Nup107/62 and/or Nup153 depletion. Fig. 6 Nup107, Nup62 , and Nup153 depletion disrupts KMT2A, EHMT2, and EZH2 occupancy at the Kcnq1ot1 ICR and imprinted gene promoters. a KMT2A, b EHMT2 and c EZH2 ChIP at the maternal and paternal Kcnq1ot1 ICR and imprinted gene promoters in control and Nup -depleted XEN cells ( n = 3 biological samples with three technical replicates per sample). The y -axis indicates total ChIP allelic enrichment levels represented as percent of input. Allelic proportions are represented as a percent of the total ChIP enrichment level. Error bars, s.e.m. ; *, significance p < 0.05 compared to the siNT control ( t test) Full size image NUPs promote cohesin interactions at paternal Kcnq1ot1 ICR Another mechanism that may alter Kcnq1ot1 imprinted domain regulation is CTCF and/or cohesin complex binding. Previous studies identified two CTCF-binding sites within the Kcnq1ot1 ICR that were bound by CTCF and the cohesin complex in mouse embryonic fibroblasts (MEFs) [2] , [43] , [44] . Thus, we investigate the relationship between CTCF, cohesin proteins, and nucleoporins at the Kcnq1ot1 domain. Next, we ruled out that nucleoporin depletion per se altered CTCF, SMC1A, or SMC3 levels in control and Nup -depleted XEN cells (Supplementary Fig. 24a, b ). As a positive control, CTCF, structural maintenance of chromosomes 1a (SMC1A), and 3 (SMC3) antibodies were validated in embryonic stem cells at the H19 ICR [2] , where strong CTCF, SMC1A, and SMC3 enrichment was observed on the maternal H19 ICR (Supplementary Fig. 25 ). To determine whether CTCF, SMC1A, and SMC3 localized at the Nup -positive enrichment sites at the Kcnq1ot1 domain, ChIP was performed using CTCF, SMC1A, and SMC3 antibodies in XEN cells. No CTCF occupancy was observed at the Kcnq1ot1 ICR and enhancer region in XEN cells (Supplementary Fig. 25b ). By comparison, SMC1A and SMC3 binding was significantly enriched at IC3 and IC4, but not at other tested sites, with preferentially cohesin binding at the paternal alleles (Fig. 7a, b ). This binding was significantly decreased upon Nup107 / Nup62 and Nup153 depletion, but not Nup98/96 depletion (Fig. 7a, b ). Fig. 7 SMC1A and SMC3 enrichment at the paternal Kcnq1ot1 ICR reduced upon nucleoporin depletion. Quantitative ChIP analysis and allelic analysis for a SMC1A and b SMC3 at positive mAb414 and NUP153 enrichment sites in control and Nup107 / Nup62 -double, Nup98/96 - (IC3, IC4 only) and Nup153 -depleted XEN cells ( n = 3 biological samples with three technical replicates per sample). Allelic proportions are represented as a percent of the total enrichment level. Error bars, s.e.m. ; *, significance p < 0.05 compared to the siNT control ( t test) Full size image To determine whether nucleoporin depletion resulted in decreased occupancy at other sites outside the Kcnq1ot1 domain, we tested SMC1A and SMC3 binding at positive and negative sites (ES cells ChIP sequencing data [45] ) within the promoters of Vim (NUP153 positive), Orai2 (NUP153, mAb414 and NUP98 positive), Shank2 (NUP153, mAb414 and NUP98 positive), as well as the Dhcr7 promoter (NUP153, mAb414, NUP98 negative site), in control and Nup -depleted cells. SMC1A and SMC3 recruitment was not altered at these sites upon nucleoporin depletion (Supplementary Fig. 26 ), indicating that SMC1A and SMC3 binding at Vim, Orai2, Shank2 , and Dhcr7 were nucleoporin-independent, whereas binding at the Kcnq1ot1 ICR was Nup107-, Nup62 -, and Nup153 -dependent. Finally, to gain an understanding of specific interactions between NUP107, NUP62, NUP153, and CTCF, SMC1A and SMC3, we performed immunoprecipitation assays using control and Nup -depleted nuclear lysates and mAb414 and NUP153 antibodies, followed by western analysis with CTCF, SMC1A, and SMC3 antibodies. We first established that NUP107/62 and NUP153 interacted with CTCF, SMC1A, SMC3 in control cells, and that these interactions were reduced in Nup107/62- and Nup153 -depleted cells (Supplementary Fig. 27 ). We next determined whether interaction with CTCF, SMC1A, and SMC3 occurred selectively through NUP107/62, and/or NUP153. In Nup107/62 -depleted cells, interactions between NUP153 and CTCF, SMC1A, and SMC3 were reduced compared to control cells (Fig. 8a ). By comparison, in Nup153 -depleted cells, mAb414 (NUP107/62) maintained CTCF, SMC1A, SMC3 interactions similar to controls (Fig. 8a ), indicating that NUP107/62 was required for NUP153 interactions with CTCF, SMC1A, and SMC3. To delineate whether these interactions were mediated via NUP107 or NUP62, NUP153 interactions were investigated in Nup107- and Nup62- depleted cells. Notably, NUP107 but not NUP62 reduced NUP153 interactions with CTCF, SMC1A, and SMC3, indicating that CTCF and cohesin interactions are mediated through NUP107 (Fig. 8b ). Fig. 8 NUP107 is required for NUP153 and NUP62 interaction with CTCF, SMC1A, and SMC3. a NUP-immunoprecipitation with NUP153 and mAb414 antibodies was performed on control (siNT) and Nup107 / 62- and Nup153 -depleted XEN nuclear lysates, following which western analysis was conducted using CTCF, SMC1A, and SMC3 antibodies ( n = 3 biological replicates). b NUP-immunoprecipitation with NUP153 antibodies was performed on Nup107- and Nup62 -depleted XEN lysates, followed by western analysis using CTCF, SMC1A, and SMC3 antibodies ( n = 3 biological replicates) Full size image In recent years, studies in mammalian cells, yeast, and Drosophila have identified roles for nucleoporins in gene regulation [22] , [23] , [27] , [28] , [46] , [47] , although the mechanistic action of nucleoporins in this regulation is not fully understood. Here, we identified a nucleoporin-dependent regulatory mechanism at the Kcnq1ot1 imprinted domain. More specifically, NUP107, NUP62, and NUP153 regulated paternal Kcnq1ot1 domain positioning at the nuclear periphery; Kcnq1ot1 ncRNA expression and volume; paternal allelic repression of multiple imprinted genes; maintenance of an active conformation at the paternal Kcnq1ot1 ICR and a repressed conformation at the paternal Osbpl5, Phlda2, Slc22a18 , Cdkn1c, Kcnq1 , and Cd81 promoters; and cohesin complex interactions at the paternal Kcnq1ot1 ICR (Supplementary Fig. 28 ). Interactions between NUP107, NUP62, and NUP153 have previously been documented in HeLa cells [35] , [37] , [48] , [49] . Investigation of various nucleoporin interactions in U2OS cells found that three of the 11 tested had the capacity to recruit other nucleoporins, which included NUP153 and NUP107 [50] . The NUP153- and NUP107-induced structure also repositioned an integrated chromatin marker from the nuclear interior to the nuclear periphery. By comparison, NUP98 possessed very limited capacity to recruit nucleoporins or target chromatin to the nuclear periphery. In keeping with this, we found that Nup107 , Nup62 , and Nup153 depletion diminished Kcnq1ot1 domain positioning at the nuclear periphery, suggesting that NUP107, NUP62, and NUP153 act at the Kcnq1ot1 ICR to tether the Kcnq1ot1 domain to the nuclear periphery. Coordinate binding of NUP107 with NUP62 and NUP153 likely mediates their regulatory role in Kcnq1ot1 ICR. Having said this, other sites within the domain maintained their NUP107/62 and NUP153 enrichment upon Nup153 depletion or Nup107 / Nup62 depletion, respectively. For example, we observed that NUP107/62 remained bound at the Osbpl5 promoter and enhancer upon Nup153 depletion. However, even when these nucleoporin interactions were maintained, the Kcnq1ot1 domain shifted away from the nuclear periphery. The most direct explanation is that NUP107/62 and NUP153 coordinately tethered the Kcnq1ot1 ICR to the nuclear periphery through the nuclear pore complex, while NUP107/62 and NUP153 binding at other regions of the domain were through an off-pore function. Recent studies have identified multiple nucleoporins (NUP62, NUP153, NUP98 and NUP50) that are present in the nucleoplasm as mobile fractions and regulate genes away from the nuclear periphery by binding their promoters [27] , [51] , [52] , [53] . Previous studies demonstrated that the Kcnq1ot1 ncRNA-coated domain is compartmentalized to the nuclear periphery or perinucleolar regions [7] , [8] , [29] , which suggests a linkage between the Kcnq1ot1 ncRNA and nuclear positioning. Here, while Nup107 , Nup62 , and Nup153 depletion displaced nuclear peripheral positioning of the paternal Kcnq1ot1 domain, the Kcnq1ot1 ncRNA remained associated with the Kcnq1ot1 domain in Nup107- , Nup62- , and Nup153 -depleted XEN cells, albeit with lower Kcnq1ot1 volumes. This suggests that the Kcnq1ot1 ncRNA per se does not regulate paternal Kcnq1ot1 domain positioning at the nuclear periphery. Alternatively, Kcnq1ot1 ncRNA coating must reach a specific threshold level to enable nuclear periphery positioning. However, the shift from random to nuclear periphery positioning of the maternal Kcnq1ot1 domain (low Kcnq1ot1 ncRNA volumes) in Nup153 -deleted cells does not support the idea of threshold levels. Previous studies found domain-wide loss of paternal allelic silencing in midgestation embryos harboring paternal deletion of the Kcnq1ot1 ICR or truncation of the paternal Kcnq1ot1 ncRNA [5] , [6] , [12] . This contrasted with our findings in Nup107- , Nup62- , and Nup153 -depleted XEN cells, where paternal alleles were reactivated at a core group of imprinted genes ( Slc22a18 , Cdkn1c , and Kcnq1 ), and at specific imprinted genes in a nucleoporin-specific manner ( Osbpl5 in Nup107 and Nup62 , Phlda2 in Nup107 , and Cd81 in Nup153 -depleted cells). One possible explanation for lack of domain-wide loss of paternal allelic silencing is that the Kcnq1ot1 ncRNA acts to coordinately regulate paternal allelic silencing of the core group of genes, while genes more distal from the Kcnq1ot1 ICR were regulated by a Kcnq1ot1 ncRNA-independent mechanism. Alternatively, Kcnq1ot1 ncRNA may operate in a gene-specific capacity across the domain. In day 14.5 placenta, Kcnq1ot1 ncRNA interactions were found at genes within ( Cdkn1c and Kcnq1 ) and outside ( Osbpl5 and Cd81 ) the core group [8] . Interactions between the Kcnq1ot1 ncRNA and PRC2 or EHMT2 could direct repressive epigenetic marks, H3K27me3 and H3K9me2, respectively, to these paternally silent genes [8] . This is supported by our data, since alterations in KMT2A, EHMT2, and EZH2 binding occurred concomitantly with changes in H3K4me3, H3K9me2, and H3K27me3 levels, respectively, at the Kcnq1ot1 ICR and paternal imprinted gene promoters upon Nup107/62 and/or Nup153 depletion. Recently, NUP153 was identified to play a role in PRC1 silencing of developmental genes in ES cells [27] . This is consistent with reactivation of the normally silent maternal Kcnq1ot1 allele upon Nup15 3 depletion. Thus, nucleoporins may interact with different macromolecular epigenetic complexes to regulate gene expression. For example, NUP107, NUP62, and NUP153 may interact with a complex containing KMT2A to enable Kcnq1ot1 ncRNA expression, while NUP153 may engage with a repressive complex to regulate maternal Kcnq1ot1 ncRNA silencing. A coordinate role for NUP107 and NUP62 has been identified at spindles and kinetochores [54] , where they may function in chromatin reorganization upon nuclear membrane reformation [23] . Our findings also point to a role for NUP107, NUP62, and NUP153 in conferring chromatin structure at the Kcnq1ot1 domain. Interactions between NUP107, NUP62, and NUP153 and the cohesin complex at the nuclear periphery on both sides of the Kcnq1ot1 promoter could enable an open chromatin configuration at the paternal Kcnq1ot1 ICR, enabling Kcnq1ot1 transcription. This is supported by reactivation of the maternal Kcnq1ot1 ncRNA allele coincident with a shift in maternal Kcnq1ot1 domain positioning at the nuclear periphery upon Nup153 depletion. Demarcation of active chromatin by NUP107, NUP62, NUP153 and cohesin may separate active chromatin at the paternal Kcnq1ot1 ICR from repressive chromatin at the paternal alleles of the core group of imprinted genes, blocking their expression. Upon Nup107 / Nup62 and Nup153 depletion, cohesin binding was reduced at the paternal Kcnq1ot1 ICR, possibly altering chromatin states at the paternal Kcnq1ot1 ICR and the core group of imprinted genes, leading to alteration in paternal allelic expression. In addition, NUP107/NUP62 binding at the Osbpl5 promoter, and NUP153 binding at the Cd81 promoter could demarcate repressive chromatin at Osbpl5 and Cd81 from active chromatin at neighboring nonimprinted genes in XEN cells. Upon Nup107 / Nup62 and Nup153 depletion, chromatin structure change at the paternal Osbpl5 and Cd81 promoters could lead them to adopt the active chromatin structure of neighboring nonimprinted genes. Thus, further investigations are required to determine the role of NUP107, NUP62, and NUP153 in regulating higher-order chromatin structure at the Kcnq1ot1 imprinted domain. Overall, dynamics of nucleoporin-mediated regulation of the Kcnq1ot1 domain highlights the complexity of epigenetic processes required to maintain imprinting across a large imprinted domain during early development. Further investigations are required to determine whether this mechanism in XEN cells is conserved in embryonic and trophoblast stem cells. The question also remains whether nucleoporins act as global imprinting regulators, operate at a subset of imprinted domains, or are specific to the Kcnq1ot1 imprinted domain. As a preliminary query, we analyzed NUP153 DAM ID-seq from ES cells, and found enrichment peaks at multiple ICRs, including Gtl2 , Snrpn , Igf2r , Peg1 and Peg10 , in addition to the at Kcnq1ot1 ICR [27] . This suggests a more generalized role for NUP153 and possibly other nucleoporins in imprinted domain regulation. Finally, identification of additional candidate epigenetic factors involved in paternal allelic silencing at the Kcnq1ot1 domain opens a new dimension of investigations into understanding imprinted domain regulation. XEN cell culture, treatments, and transfection CASTX Cdkn1c Δneo R B6 XEN stem cells were generated by crossing a Mus musculus casteneus (CAST) female (Jackson Laboratory) to a C57BL/6J (B6) male carrying a targeted mutation of the Cdkn1c gene in which exons 1 and 2 were replaced by the PGK-Neomycin resistance cassette ( Cdkn1c Δneo R ) [18] (Jackson Laboratory). B6XCAST XEN cells were generated from crosses between C57BL/6J (B6) female and CAST males. Briefly, embryos were collected at embryonic day E3.5 as late morula or blastocyst and plated on mitomycin C (Sigma, M4287)-treated mitotically inactive MEFs in XEN cell medium [17] (RPMI (Sigma, R0883) supplemented with 50 μg/mL penicillin/streptomycin, 1 mM sodium pyruvate, 100 μM β-mercaptoethanol, 2 mM l -glutamine, 15% hyclone ESC grade FBS). On day 2, blastocysts hatched and attached to the plate. On days 3–4, small outgrowths were formed for each embryo. XEN cell medium was replaced every 2 days until XEN cell colonies appeared, which were further passaged on mitomycin C mitotically inactive MEFs. CASTX Cdkn1c Δneo R B6 XEN stem cells were genotyped for paternal Cdkn1c Δneo R allele using p57neo primers (Supplementary Table 1 ). Experiments were performed in compliance with guidelines set by the Canadian Council for Animal Care, and the policies and procedures approved by the University of Western Ontario Council on Animal Care. XEN cells were cultured on a gelatin-coated (EmbryoMax ® 0.1% Gelatin Solution, Millipore, ES-006-B), feeder-free environment prior to experiments to avoid feeder contamination [1] . Three wild-type B6XCAST XEN cell lines, which were produced from different embryos, with 2–5 technical replicates per line, were used for each experiment, except for the DNA methylation analyses, where two biological replicates were analyzed. Where specified, cells were synchronized in G1 phase by treatment with 2 mM hydroxyurea (Sigma, H8627) for 12 h followed by siRNA transfection. Cells were transfected with 10 nmol of siRNAs with 3.6 μL siPepMute™ siRNA Transfection Reagent (SignaGen, SL100566) in 100 μL of 1× transfection buffer. Fresh XEN medium was added 2 h before transfection. 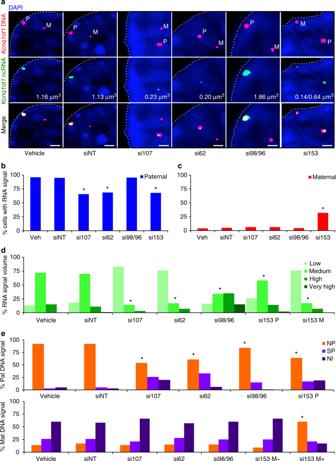Fig. 2 Nucleoporin depletion disruptedKcnq1ot1ncRNA volume andKcnq1ot1domain positioning at the nuclear periphery.aRepresentative confocal nuclear images displayingKcnq1ot1DNA (magenta)Kcnq1ot1ncRNA (cyan) and DAPI staining (blue) for G1-synchronized control andNup-depleted XEN cells (n= 4; cell number = 109–123); upper panel, DNA FISH; middle panel, RNA FISH; lower panel, merge; M maternal domain, P paternal domain; white dashed line denotes nuclear rim. In these images, red and green fluorescence was converted to magenta and cyan.b,cPercent of cells with paternal or maternalKcnq1ot1ncRNA signals.dPercent of cells withKcnq1ot1ncRNA signal volume; low, 0–0.7 μm3; medium, 0.7–1.4 μm3; high, 1.4–2.1 μm3; very high, >2.1 μm3.eDistance of the paternal and maternalKcnq1ot1domain from the nuclear membrane in control andNup-depleted XEN cells. The maternalKcnq1ot1domain was randomly positioned within the nucleus (expected nuclear periphery (NP) 15%; subnuclear periphery (SP) 30%; nuclear interior (NI) 60%), except forNup153-depleted cells with aKcnq1ot1ncRNA signal (si153 M+). For these analyses, cells with no RNA but detectable DNA FISH signals were included, while those lacking DNA signals were excluded. NP, 0–0.5 μm; SP, 0.5–1.5 μm; NI, 1.5–4 μm; error bars, s.e.m.; *, significancep< 0.05 compared to vehicle control (ttest); WT wild type, Veh vehicle, siNT nontargeting siRNA, si107Nup107siRNA, si62Nup62siRNA, si98/96Nup98/96siRNA, si153Nup153siRNA, si153 M-Nup153-depleted cells without aKcnq1ot1ncRNA signal; scale bar, 1 μm;n= 4; cell count number = 109–123 siRNA sequences are listed in Supplementary Table 2 . Recombinant virus production and lentiviral transduction A library of shRNAs targeting 250 different epigenetic factors used in this experiment was previously described [17] . Transduction of shRNAs into XEN cells was modified from ref. [17] . Briefly, shRNA vectors and lenticlass plasmids encoding Vesicular stomatitis virus glycoprotein pseudotype (plasmid pMDG) and Psi (pPsi) packaging elements were transfected into 10 cm dishes of HEK293 cells (ATCC ® , CRL-3216 ™ ) using Lipofectamine 2000 (Invitrogen, 11668027). The ratio of plasmids transfected was 2.3 μg shRNA vectors, 1.0 μg pMDG, and 1.7 μg of pPsi. Medium was changed 6 h later. Viral-containing media was harvested and filtered (0.45 µm pore) 72 h post-transfection and added to freshly trypsinized XEN cells along with 1× polybrene (Sigma, TR-1003-G) into 1× 6-well plates (Corning, C3506). XEN cell media was changed 48 h later. Low levels of infection were necessary to ensure single viral integration per cell and was verified using flow cytometry. For flow cytometry analysis, cells were washed twice with 1× PBS (Sigma, D8537) and trypsinized (Sigma, T4174) into single cell suspensions. Cells were pelleted and resuspended in 10% FBS in 1× PBS solution followed by analysis on Beckman Coulter Epics XL-MCL Flow Cytometer. XEN cells were selected for viral integration with 1 μg/mL puromycin (Sigma, P8833). shRNA containing XEN cells were moved to 8 × 10 cm dishes (Corning, 430167) and selected for loss of silencing of the Cdkn1c Δneo allele with 50–200 μg mL −1 neomycin (Sigma, G8168). While still under neomycin selection, XEN cells were replated at a lower density onto 15 cm dishes until individual colonies were formed. Individual colonies were picked and transferred over to 24-well dishes (Corning, C3527), and then underwent a second round of neomycin selection. DNA and RNA isolation, cDNA preparation and PCR amplification DNA of surviving colonies from the lentiviral screen was isolated using Qiagen DNeasy Blood & Tissue Kit (Qiagen, 69504) and PCR amplification was performed for the hairpin region inside the shRNA construct with primers targeting the lentiviral sequence [17] . RNA was isolated using PureLink ® RNA Mini Kit (Life Technologies, 12183018A), QuickRNA TM MicroPrep (Zymo Research, R1050) or RNeasy Plus Mini Kit (Qiagen, 74134) according to the manufacturers’ instructions. Before cDNA preparation, total RNA was subjected to DNase I (Life Technologies, 18068015) treatment as described [1] . cDNA was prepared using ProtoScript ® II Reverse Transcriptase (NEB, M0368X) as per instructions with oligodT 23 (Sigma, O4387) and Random Primers (Life Technologies, 48190011). cDNA was treated with RNaseA (Roche, 10109142001) after preparation to remove residual RNA. PCR was performed on CFX1000 and MJ Research Thermocyclers (Bio-Rad). Quantitative PCR analysis Quantitative (q) PCR was performed as described [1] . Briefly, qPCR was performed using iQ SYBR Green Supermix (Bio-Rad, 1708880) or SensiFAST TM SYBR ® No-ROX Kit (Bioline, BIO-98005) on an MJ Thermocycler Chromo4 Real-time PCR system (Bio-Rad, CFB-3240) or a CFX-96™ Real-time system (Bio-Rad, 185-5096). For gene expression analysis, data were analyzed using the 2ΔΔCT method [55] . For ChIP, qPCR data analysis was performed as described [56] . Supplementary Table 1 lists primers, annealing temperatures, and amplicon sizes. Droplet digital PCR allelic expression analysis Droplet digital PCR (ddPCR) probes and primers were designed following Bio-Rad’s guidelines for ddPCR assays. Single nucleotide polymorphisms (SNPs) between C57BL/6 and CAST genomes in target genes were assessed with OligoAnalyzer 3.1 [57] . SNPs that generated the greatest difference in melting temperature ( T m ) between the alleles, in either forward and reverse compliment strands, were selected as the probe target. Primers and probes were designed using Primer3plus [58] , RealTimeDesign™ software (BIOSEARCH Technologies) [59] , OligoAnalyzer 3.1 [57] , or advice from IDT. For primer design, a target T m was set for ~60 °C with each primer being within ~2 °C of each other. When possible, amplicon size was kept between 80 and 200 bp, but larger amplicons were possible with optimized PCR amplification programs. Amplicons with repeats of Gs and Cs longer than three bases, especially at the 3′-end, were avoided. For probe design, the target length was set to 11–22 bp, and where possible the SNP was centered within the probe. Caution was taken to ensure that a G nucleotide was not at the 5′ of start of probe. A probe T m of 3–10 °C higher than the primer pairs was required. Shorter probes incorporated locked-nucleic acids (LNA) to achieve the probe target T m . EXIQON LNA Oligo Tm Prediction [60] was used to predict T m changes from adding LNAs. Increased probe T m were also achieved with longer probes, in this case a ZEN-quencher (Integrated DNA Technologies; IDT) was added to the center of the probe to dual-quench the fluorophores. Following probe design, a T m difference of ≥3 °C between the probes was confirmed using OligoAnalyzer 3.1 [57] . Probes for Cd81, Cdkn1c, Th , and Tssc4 were designed by IDT. All probes were synthesized by IDT with FAM or HEX fluorophores quenched by Iowa Black FQ. Primer and probe sequences are listed in Supplementary Table 1 . For ddPCR sample preparation, RNA was extracted using the RNeasy Plus Mini Kit (Qiagen, 74134) according to the manufacturers’ instructions. RNA concentrations were determined using Qubit ® 3.0 Fluorometer (Life Technologies, Q33216), Qubit RNA BR Assay Kit (ThermoFisher Scientific, Q10210) and Qubit RNA HS Assay Kit (ThermoFisher Scientific, Q32852). Before cDNA preparation, total RNA was subjected to DNase I (Life Technologies, 18068015) treatment. cDNA was prepared using ProtoScript II Reverse Transcriptase (NEB, M0368X), oligo(dT) 23 (Sigma, O4387) and Random Primers (Life Technologies, 48190011). cDNA was treated with RNaseA (Roche, 10109142001) after preparation to remove residual RNA. For each gene, ddPCR master mixes were made for a reaction final volume of 22 µL, containing; 2–4 µL cDNA, 1 µL of primers each (250 nM), 1 µL of probes each (FAM, HEX 250 nM), 11 µL ddPCR Supermix for Probes (no dUTP) (Bio-Rad,1863024), and 3–5 µL DNAse-RNAse free UltraPure dH 2 0 (Invitrogen, 10977-015). Each reaction was loaded into a 96-well plate (Bio-Rad, 12001925), sealed using a foil heat seal (Bio-Rad, 1814040) and placed into a PX1 PCR Plate Sealer at 180 °C for 5 s. Sealed plates were loaded into the AutoDG (Bio-Rad, 1864100) for droplet generation. Droplets were loaded into a new 96-well plate (Bio-Rad, 12001925) and sealed using a foil heat seal (Bio-Rad, 1814040). Droplet digital PCR (ddPCR) was performed on a deep well CFX1000 (Bio-Rad,1851197). Optimal annealing temperature for each primer/probe set is listed in Supplementary Table 1 . For most genes, a standard ddPCR program of 10 min at 95 °C, 40 cycles of 94 °C for 30 s and annealing temperature for 60 s, and a final cycle of 10 min at 98 °C. For Cdkn1c , that has a longer amplicon, an additional step was added to the program to enhance fluorophore release (10 min at 95 °C, 40 cycles of 94 °C for 30 s and 60 °C for 60 s, 10 cycles of 94 °C for 30 s and 50 °C for 60 s, and a final cycle of 10 min at 98 °C). Following PCR, the droplets were read on the QX200 (Bio-Rad, 1864100), set for detecting absolute levels of FAM/HEX probe fluorophores. Each positive droplet in a ddPCR assay represents a template molecule in the sample, allowing for absolute quantification of allelic expression. Using Quantasoft Analysis Pro 1.0.596 (Bio-Rad), droplets from FAM and HEX identified alleles were selected using the 1D and 2D Amplitude tool. Any FAM/HEX double-positive droplets represent doublets containing both alleles, and these were eliminated from analysis. Copies per μL values that were determined from Quantasoft Analysis Pro were converted to copies per μg and plotted using BoxPlotR [61] . RNA/DNA FISH, immunocytochemistry and confocal microscopy Kcnq1ot1 RNA/DNA FISH probe was generated using a 32-kb fosmid Wl1-2505B3 in the Kcnq1 intronic region (BACPAC Resources Center at the Children’s Hospital Oakland Research Institute, Oakland, CA) using the BioPrime DNA labeling System (ThermoFisher Scientific, 18094011) with fluorescein-12-dUTP (Roche, 11373242910) and Biotin-16-dUTP (Roche, 11093070910) for RNA FISH, and Cy5-UTP (GE Healthcare, 45001239) for DNA FISH as described [1] . For RNA FISH, cells seeded on coverslips (VWR, 48380046) in 12-well plates (Corning, C3512) were fixed, dehydrated in a series of 25, 50, 75, and 100% ethanol followed by hybridization with RNA-FISH probes in 100% molecular grade formamide (VWR, 97062-006) as described [1] . Briefly, following overnight incubation at 37 °C in a formamide sealed hybridization chamber, coverslips were carefully washed in 4× SSC and 2× SSC (ThermoFisher Scientific, AM9763) at 37 °C for 5 min three times each. All washes were done in 12-well tissue culture plates. Coverslips were incubated with primary antibody in blocking buffer (20× SSC, 10% Tween-20 (Sigma, P9416), 10% Skim Milk) at 37 °C for 1 h in the dark, then washed three times with 4× SSC (37 °C) with agitation. Next, coverslips were incubated with the secondary antibody in blocking buffer at 37 °C in the dark for 1 h, then washed three times with 4× SSC and two times with 2× SSC buffers at 37 °C with continuous agitation, 5 min each. The final wash was done in 1× SSC for 5 min. SSC buffer was made fresh from 20× stock and pre-heated to 42 °C during the washes. Coverslips were mounted on glass slides with Vectashield DAPI (antifade mounting medium, Vector labs, H-1000) and stored in the dark for a few hours or overnight at 4 °C. For DNA/RNA FISH, DNA FISH was first performed as described [33] followed by RNA FISH. Briefly, fixed cells were rinsed with 1× PBS and dehydrated in a series of ethanol washes. DNA was denatured by incubating the coverslips with 70% formamide in 2× SSC at 85 °C for 20 min. Coverslips were quickly washed with 2× SSC and hybridized with DNA FISH probes overnight at 37 °C in a sealed formamide chamber (sealed with parafilm). Next day, excess probe was washed with pre-warmed (42 °C) 4× SSC and 2× SSC buffer three times each. Coverslips were then incubated with RNA FISH probe. RNA FISH was performed as described above. For immunocytochemistry assays, XEN cells were seeded on gelatin-treated coverslips in 12-well plates. Cells were permeabilized with sequential transfers into ice-cold cytoskeletal extraction buffer (CSK) for 30 s, ice-cold CSK containing 0.25% Triton X-100 for 45 s and ice-cold CSK for 30 s. Following CSK treatment, cells were fixed in freshly prepared 4% paraformaldehyde (Sigma, P6148) at room temperature for 10 min, washed twice in 1× PBS and stored in 70% ethanol for up to a month. Cells were washed three times in 1× PBS for 5 min each followed by incubation in primary antibody in 5% skim milk for 1 h at room temperature, washed three times with 1× PBS followed by incubation with secondary antibody. Cells were then washed three times with 1× PBS, stained with DAPI and mounted on glass slides for confocal microscopy. 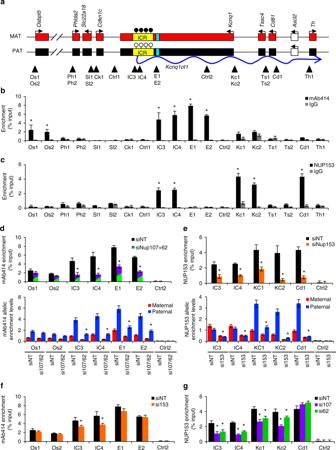Fig. 3 NUP107/62 and NUP153 interaction with theKcnq1ot1ICR, and theOsbpl5, Kcnq1, Cd81promoters.aTheKcnq1ot1domain with regions of analysis (arrowheads) at theKcnq1ot1ICR, IC3, IC4; enhancer element, E1, E2; imprinted gene promoters; Os1, Os2, Ph1, Ph2, Sl1, Sl2, Ck1, Kc1, Kc2, Ts1, Ts2, Cd1, Th1; and negative control sites, Ctrl1, Ctrl2. Quantitative ChIP analysis usingbmAb414 antibodies andcNUP153 antibodies in wild-type XEN cells at regions across the domain, respectively (n= 3 biological samples with four technical replicates per sample). Quantitative allelic analysis fordmAb414 andeNUP153 in siNT- and nucleoporin-depleted XEN cells. Allelic proportions are represented as percent of the total enrichment levels (n= 3 biological samples with four technical replicates per sample).fQuantitative ChIP analysis using mAb414 antibodies was performed in control andNup153-depleted XEN cells at sites of NUP153 enrichment (n= 3 biological samples with three technical replicates per sample).gQuantitative ChIP analysis using NUP153 antibodies was performed in control andNup107-andNup62-depleted cells at sites of mAb414 (NUP107/62) enrichment (n= 3 biological samples with three technical replicates per sample). Error bars, s.e.m.; *, significancep< 0.05 compared to the IgG or siNT control (ttest) Supplementary Table 3 lists antibody dilutions. Coverslips were imaged using z-stacks on a FluoView FV1000 coupled to an IX81 motorized inverted system (Olympus). For DNA and RNA FISH, signal volume was measured in Volocity (PerkinElmer) with z-stacks intensity-based thresholding (µm 3 ), while distances of DNA FISH signal centroid from the nuclear rim were calculated to determine domain positioning (µm) (ImageJ). Western blot analysis and immunoprecipitation assay Cytoplasm and nuclear protein extracts were isolated using cytoplasm extraction buffer and nuclear extraction buffer using the NE-PER Nuclear and Cytoplasmic Extraction Kit (ThermoFisher Scientific, 78833) followed by western blot analysis as described [17] [62] . Briefly, protein samples were quantified using the Bradford assay, Nanodrop or Qubit protein concentration determination assay. Typically, 20–30 μg of protein was separated on an 8–12% SDS-PAGE (Bio-Rad, Bulletin 6201) gel or any kD™ Mini-PROTEAN ® TGX™ Precast Protein Gels (Bio-Rad, 4569033), transferred to PVDF membrane (Bio-Rad, 1620177) or Trans-Blot ® Turbo™ Mini PVDF Transfer Packs (Bio-Rad, 1704156), blocked for 1 h in 5% skim milk in 1× TBST (1× TBS (Bio-Rad, 1706435) with 0.1% Tween-20, (Sigma, P9416)), incubated with primary antibody in 5% skim milk as described in Supplementary Table 3 followed by three washes of 1× TBST for 7 min each. Blots were next incubated with secondary antibody in 5% skim milk followed by detection using chemiluminescence reaction with Clarity Western ECL Substrate (Bio-Rad, 1705060). For list of antibodies and dilutions see Supplementary Table 3 . Uncropped scans of western blots presented in the main figures are provided in Supplementary Figs. 30 – 38 . Protein co-immunoprecipitation was performed using Dynabeads Protein G (Invitrogen, 10004D) as per the manufacturer’s instructions. Briefly, 50 μg of nuclear lysates obtained from XEN cells using the NE-PER Nuclear and Cytoplasmic Extraction Kit (ThermoFisher Scientific, 78833) were incubated with the respective antibody, 2 μL RNase A (Roche, 10109142001), 2 μL DNase I (Life Technologies, 18068015), and 4 μL protease inhibitor (Sigma, P8340) as described in Supplementary Table 3 overnight at 4 °C. Samples were then incubated with Dynabeads protein G (Invitrogen) for 1 h at 4 °C. Immunoprecipitates were washed three times with 200 μL of 0.1% Tween-20 in 1× PBS, eluted in 1× Laemmli buffer (Bio-Rad, 1610747) and resolved on 10–12% SDS-PAGE followed western blot analysis as described above. Chromatin immunoprecipitation (ChIP) assay ChIP was performed as described with modifications for siRNA depletions [56] . Equal numbers of cells were collected from control and siRNA treatment groups (~0.5–1.2 million cells). 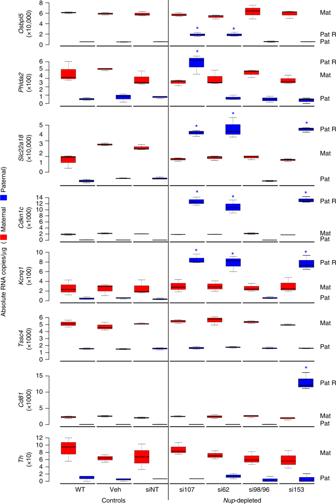Fig. 4 Nup107, Nup62, andNup153depletion reactivate a subset of paternal alleles at theKcnq1ot1domain. Absolute allelic transcript abundance of imprinted genes determined by droplet digital PCR in control andNup-depleted XEN cells, as a measure of RNA copies µg−1(n= 3 biological samples). Center lines, medians; box limits, 25th and 75th percentiles as determined by R software; whiskers, 1.5 times the interquartile range from 25th and 75th percentiles; Mat, maternal; Pat, paternal; Pat R, reactivated paternally silent allele; *, significancep< 0.05 compared to the siNT control (ttest). Error bars, s.e.m. Approximately 40,000 cells were used per ChIP reaction. Briefly, cells were cross-linked in freshly prepared 1% formaldehyde final concentration for 6 min, quenched in 1.25 M glycine at room temperature for 5 min, followed by wash in 200 μL 1× PBS. Pellets were resuspended in 200 μL of cytoplasm extraction buffer (10 mM HEPES (pH 7.6), 60 mM KCl, 1 mM EDTA, 1 mM DTT, 0.075% NP40, 1 mM PMSF) and incubated on ice for 5 min followed by spin at 3000 rpm at 4 °C for 4 min. Nuclear pellets were lysed by resuspension in 100 μL 1% SDS buffer for 10 min on ice, followed by addition of 100 μL 1× TE, 3μL of proteinase inhibitor (Sigma, P8340) and then sonicated (Diagenode, B01060001 or Covaris M220) to shear chromatin into 100–400 bp fragments, followed by immunoprecipitation. Frozen cross-linked chromatin lysates were stored at −80 °C. Protein G Dynabeads (8 μL, Life Technologies) were washed three times with ChIP dilution buffer (0.1% SDS, 1% Triton X-100, 2 mM EDTA, 20 mM Tris pH 8.1, 500 mM NaCl). Magnetic beads were bound with 1.5–4 μg of antibody at 4 °C for 1 h followed by incubation with precleared chromatin lysate (equivalent to 40,000 cells) for 3 h to overnight (as specified in antibody table). Chromatin lysate (10 μL) was saved as Input. Beads were washed at 4 °C once with 200 μL of Low Salt Buffer (0.1% SDS, 1% Triton X-100, 2 mM EDTA, 20 mM Tris pH 8.1, 150 mM NaCl) for 5 min, followed by two washes with 200 μL of High Salt Buffer (0.1% SDS, 1% Triton X-100, 2 mM EDTA, 20 mM Tris pH 8.1, 500 mM NaCl) for 5 min each. Beads were next washed once with 200 μL 1× TE Wash Buffer (10 mM Tris pH 8.1, 1 mM EDTA) at 4 °C for 5 min. DNA was eluted off the beads by incubation at 65 °C for 1 h with constant shaking in 200 μL of elution buffer (1% SDS,100 mM NaHCO 3 ). 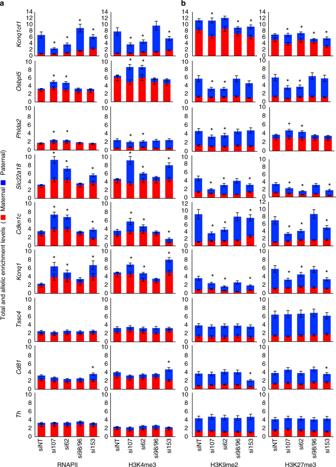Fig. 5 Nup107, Nup62, andNup153depletion disrupts RNAPII enrichment and histone modifications at theKcnq1ot1ICR and imprinted gene promoters.aRNAPII and H3K4me3 ChIP at the maternal and paternalKcnq1ot1ICR and imprinted gene promoters in control andNup-depleted XEN cells (n= 3;n= 3 technical replicates).bH3K9me2 and H3K27me3 ChIP at the maternal and paternalKcnq1ot1ICR and imprinted gene promoters in control andNup-depleted XEN cells (n= 3 biological samples with three technical replicates per sample). They-axis indicates total and allelic ChIP enrichment levels represented as percent of input. Allelic proportions are represented as a percent of the total ChIP enrichment level. Error bars, s.e.m.; *, significancep< 0.05 of paternal/maternal levels compared to the siNT paternal/maternal control (ttest) To purify eluted DNA, RNA was degraded by addition of 1 μL of 1 μg/μL RNase A (Roche) with an incubation at 37 °C for 1 h. Protein was degraded by addition of 4 μL of 10 mg/mL proteinase K (Sigma) with an incubation at 55 °C for 2 h. Following ChIP, DNA extraction was performed using Chelex beads (Bio-Rad, 1421253), ChIP DNA Clean & Concentrator TM (Zymo Research, D5201) or QIAquick PCR Purification Kit (Qiagen, 28104). ChIP-qPCR assays were performed using iQ SYBR Green Supermix (Bio-Rad, 1708880) and SensiFAST TM SYBR ® No-ROX Kit (Bioline, BIO-98005) on an MJ Thermocycler Chromo4 Real-time PCR system or a CFX-96 Real-time system (Bio-Rad) under the following conditions: 95 °C for 5 min followed by 40 cycles of 95 °C for 10 s, annealing (for temperature see Supplementary Table 1 ) for 20 s, 72 °C for 30 s, followed by plate reading. Lastly, a final melting curve was generated from 55 to 95 °C in increments of 1 °C. Enrichment levels (percent input) were calculated 100×(2^[ΔCt Input − ΔCt Input ] − [ΔCt Input − ΔCt Ab ])/25. Supplementary Table 3 lists antibody concentration. Data are represented as total enrichment (percent input) or allelic enrichment (calculated as total enrichment × allelic enrichment ratio). Statistical analysis For statistical analysis, two-tailed Student’s t test was performed on mean values. 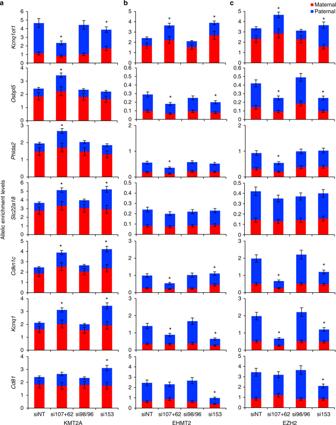Fig. 6 Nup107, Nup62, andNup153depletion disrupts KMT2A, EHMT2, and EZH2 occupancy at theKcnq1ot1ICR and imprinted gene promoters.aKMT2A,bEHMT2 andcEZH2 ChIP at the maternal and paternalKcnq1ot1ICR and imprinted gene promoters in control andNup-depleted XEN cells (n= 3 biological samples with three technical replicates per sample). They-axis indicates total ChIP allelic enrichment levels represented as percent of input. Allelic proportions are represented as a percent of the total ChIP enrichment level. Error bars, s.e.m.; *, significancep< 0.05 compared to the siNT control (ttest) Treatment samples were compared to controls. 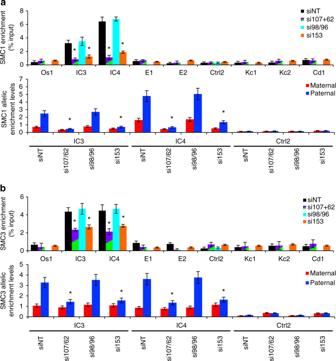Fig. 7 SMC1A and SMC3 enrichment at the paternalKcnq1ot1ICR reduced upon nucleoporin depletion. Quantitative ChIP analysis and allelic analysis foraSMC1A andbSMC3 at positive mAb414 and NUP153 enrichment sites in control andNup107/Nup62-double,Nup98/96- (IC3, IC4 only) andNup153-depleted XEN cells (n= 3 biological samples with three technical replicates per sample). Allelic proportions are represented as a percent of the total enrichment level. Error bars, s.e.m.; *, significancep< 0.05 compared to the siNT control (ttest) 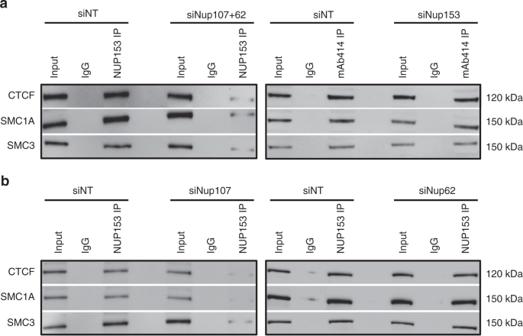Fig. 8 NUP107 is required for NUP153 and NUP62 interaction with CTCF, SMC1A, and SMC3.aNUP-immunoprecipitation with NUP153 and mAb414 antibodies was performed on control (siNT) andNup107/62-andNup153-depleted XEN nuclear lysates, following which western analysis was conducted using CTCF, SMC1A, and SMC3 antibodies (n= 3 biological replicates).bNUP-immunoprecipitation with NUP153 antibodies was performed onNup107-andNup62-depleted XEN lysates, followed by western analysis using CTCF, SMC1A, and SMC3 antibodies (n= 3 biological replicates) A p value less than 0.05 was considered to be significant. Data availability All data generated or analyzed during this study are included in this published article (and its supplementary information files). Data supporting the findings of this manuscript are available from the corresponding author upon reasonable request.